Muscle-derived stem/progenitor cell dysfunction limits healthspan and lifespan in a murine progeria model With ageing, there is a loss of adult stem cell function. However, there is no direct evidence that this has a causal role in ageing-related decline. We tested this using muscle-derived stem/progenitor cells (MDSPCs) in a murine progeria model. Here we show that MDSPCs from old and progeroid mice are defective in proliferation and multilineage differentiation. Intraperitoneal administration of MDSPCs, isolated from young wild-type mice, to progeroid mice confer significant lifespan and healthspan extension. The transplanted MDSPCs improve degenerative changes and vascularization in tissues where donor cells are not detected, suggesting that their therapeutic effect may be mediated by secreted factor(s). Indeed, young wild-type-MDSPCs rescue proliferation and differentiation defects of aged MDSPCs when co-cultured. These results establish that adult stem/progenitor cell dysfunction contributes to ageing-related degeneration and suggests a therapeutic potential of post-natal stem cells to extend health. A universal characteristic of ageing is the loss of regenerative capacity leading to an impaired ability to respond to stress and, therefore, increased morbidity and mortality [1] . This has led to the hypothesis that ageing is caused, in part, by the loss of functional adult stem cells necessary for tissue regeneration [2] , [3] . Indeed, mice greater than two years of age have a significant reduction in the number and proliferative capacity of neural stem cells [4] , [5] and male germline stem cells [6] , [7] . In contrast, with ageing, haematopoietic stem cell (HSC) numbers are preserved but their function is lost [8] , [9] . Muscle satellite cells also lose stem cell properties with ageing, but their abundance in old age remains controversial [10] , [11] , [12] , [13] . Ageing-related changes in bone-marrow-derived mesenchymal stem cells (MSCs) include loss of proliferation and differentiation potential, increase in senescence and loss of capacity to form bone in vivo [14] , [15] . Similarly, MSCs derived from the bone marrow of patients with Hutchinson–Gilford progeria syndrome, a disease of dramatically accelerated ageing, are defective in their ability to differentiate [16] . Adipose-derived multipotent cells show an age-dependent loss of self-renewal capacity and an increased propensity for adipogenesis [17] . Despite this extensive evidence for adult stem cell decline with ageing, it is not known whether old stem cells contribute to ageing-related degenerative changes or are merely a biomarker of it. Given that ageing-related degenerative changes are universal in the musculoskeletal system [18] , [19] , [20] , we investigated the impact of ageing on murine muscle-derived stem/progenitor cells (MDSPCs). MDSPCs are multipotent cells isolated from postnatal skeletal muscle through an established preplate technique [21] , [22] . They have a capacity for long-term proliferation, are resistant to oxidative and inflammatory stress, show multilineage differentiation and self-renew, induce neovascularization, and stimulate regeneration of bone, skeletal and cardiac muscles [21] , [23] , [24] , [25] . These cells likely reside in the perivascular niche [26] . These characteristics raise the possibility that the loss of MDSPCs or related perivascular progenitor cells could contribute to sarcopenia, osteoporosis [27] , [28] and other degenerative diseases associated with ageing. Here we examine MDSPC function in natural ageing and a mouse model of a human progeria. XFE progeroid syndrome is caused by mutations in XPF (xeroderma pigmentosum complementation group F) and characterized by dramatically accelerated ageing of the epidermal, haematopoietic, endocrine, hepatobiliary, renal, nervous, musculoskeletal and cardiovascular systems [29] . XPF encodes one subunit of an endonuclease that together with its essential binding partner ERCC1 (excision repair cross complementation group 1) participates in numerous DNA repair mechanisms [30] . XFE progeroid syndrome was modelled in the mouse by mutation of the mErcc1 locus to titrate expression of ERCC1–XPF [31] , [32] . Ercc1 −/− mice with undetectable levels of ERCC1–XPF have a severely reduced lifespan of 1 month (mth) [29] , [30] , [32] while Ercc1 −/Δ mice, expressing 10% of the normal level of ERCC1–XPF have a lifespan of 7 mths (refs 30 , 32 ). Both strains faithfully mimic the systemic accelerated ageing of XFE progeroid syndrome and demonstrate a highly significant correlation with naturally aged mice at the level of histopathology, pathophysiology and genome-wide transcriptional reprogramming [30] , [32] , [33] , [34] . Our results indicate that MDSPC function is adversely affected with accelerated and natural ageing. This dysfunction directly contributes to ageing-related degenerative changes since transplantation of functional MDSPCs was sufficient to extend healthspan and lifespan of progeroid mice. Furthermore, we provide evidence that the therapeutic effect of MDSPCs may be mediated by secreted factors that act systemically. Loss of stemness properties with ageing MDSPCs are slowly adhering cells isolated from skeletal muscle and enriched through a preplate technique [21] , [22] . Previously, we reported isolating these multipotent cells from young (3-week (wk)-old) mice [22] , [35] . To determine whether MDSPCs could also be isolated from adult and old mice, we followed the same preplate technique, and the resulting cells were analysed for expression of stem/progenitor cell markers (CD34, Sca-1). Cells isolated from skeletal muscle of young (3-wks), adult (19-wks), and old wild-type (WT) (2-years (yrs)) mice through this technique expressed CD34 and Sca-1 ( Fig. 1a ), establishing that MDSPCs could be isolated from mice of all ages. Although expression of CD34 appeared mildly attenuated in the older cell populations, Sca-1, which is a more stable marker of MDSPCs [36] , was similarly expressed in all three populations. Furthermore, MDSPCs isolated from adult WT mice showed multilineage differentiation ( Fig. 1b ). 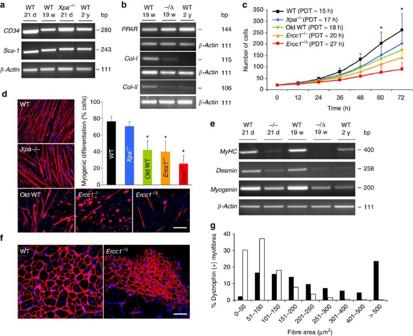Figure 1: Measuring MDSPC proliferation, differentiation, and regenerative potential. (a) rtPCR to measure stem/progenitor cell markers CD34 and Sca-1 in MDSPCs isolated from muscle of mice at various ages. Shown is a representative image from analysis of 3–4 independent MDSPC populations per genotype/age at passage 23–25. (b) rtPCR to measure differentiation markers. Peroxisome proliferator-activated receptor (PPAR) is an adipocyte marker; collagen 1 (Col-1) is an osteocyte marker; collagen-2 (Col-2) is a chondrocyte marker. β-Actin was the loading control. Shown is a representative image from analysis of three independent MDSPC populations of each genotype/age. (c) Proliferation of MDSPCs measured by live-cell imaging. Plotted are the average number of cells at each time point calculated from 3–4 populations per genotype ±s.d. (*P<0.05, Tukey's test). Average PDT was calculated from analysis of 40 images per time point. (d) Representative images ofin vitromyogenic differentiation. Cells were immunostained for the terminal differentiation marker, f-MyHC (red). Scale bar=100 μm. Quantification of myogenic differentiation was calculated as the fraction of cells (DAPI, blue) expressing f-MyHC (red) from 3–4 cell populations per genotype ±s.d; *P<0.001 relative to young WT-MDSPCs (black bar), Kruskal–Wallis ANOVA on ranks. (e) rtPCR to measure expression of the terminal differentiation markers, MyHC, desmin, and myogenin, after myogenic differentiation of MDSPCs isolated from mice of various genotypes/ages. Shown is a representative image from 3 MDSPC populations tested per group. (f) Representative image of gastrocnemius muscle sections from dystrophic mice 14 days post-injection of WT orErcc1−/ΔMDSPCs to test myogenic differentiationin vivo. The sections were immunostained for dystrophin (red) to identify myofibres from donor cells. Scale bar=100 μm. (g) Quantification of the donor myofibre area in dystrophic mice transplanted with WT-MDSPCs (black bars) or MDSPCs fromErcc1−/Δmice (white bars). Plotted is the average number of myofibres of each size range calculated from >2,000 fibres analysed permdx/SCID mouse (n=8) treated with 2 independent MDSPC populations per genotype. (P<0.001, for all distribution ranges except 101–150; Mann–Whitney rank sum test). Figure 1: Measuring MDSPC proliferation, differentiation, and regenerative potential. ( a ) rtPCR to measure stem/progenitor cell markers CD34 and Sca-1 in MDSPCs isolated from muscle of mice at various ages. Shown is a representative image from analysis of 3–4 independent MDSPC populations per genotype/age at passage 23–25. ( b ) rtPCR to measure differentiation markers. Peroxisome proliferator-activated receptor (PPAR) is an adipocyte marker; collagen 1 (Col-1) is an osteocyte marker; collagen-2 (Col-2) is a chondrocyte marker. β-Actin was the loading control. Shown is a representative image from analysis of three independent MDSPC populations of each genotype/age. ( c ) Proliferation of MDSPCs measured by live-cell imaging. Plotted are the average number of cells at each time point calculated from 3–4 populations per genotype ±s.d. (* P <0.05, Tukey's test). Average PDT was calculated from analysis of 40 images per time point. ( d ) Representative images of in vitro myogenic differentiation. Cells were immunostained for the terminal differentiation marker, f-MyHC (red). Scale bar=100 μm. Quantification of myogenic differentiation was calculated as the fraction of cells (DAPI, blue) expressing f-MyHC (red) from 3–4 cell populations per genotype ±s.d; * P <0.001 relative to young WT-MDSPCs (black bar), Kruskal–Wallis ANOVA on ranks. ( e ) rtPCR to measure expression of the terminal differentiation markers, MyHC, desmin, and myogenin, after myogenic differentiation of MDSPCs isolated from mice of various genotypes/ages. Shown is a representative image from 3 MDSPC populations tested per group. ( f ) Representative image of gastrocnemius muscle sections from dystrophic mice 14 days post-injection of WT or Ercc1 −/Δ MDSPCs to test myogenic differentiation in vivo . The sections were immunostained for dystrophin (red) to identify myofibres from donor cells. Scale bar=100 μm. ( g ) Quantification of the donor myofibre area in dystrophic mice transplanted with WT-MDSPCs (black bars) or MDSPCs from Ercc1 −/Δ mice (white bars). Plotted is the average number of myofibres of each size range calculated from >2,000 fibres analysed per mdx /SCID mouse ( n =8) treated with 2 independent MDSPC populations per genotype. ( P <0.001, for all distribution ranges except 101–150; Mann–Whitney rank sum test). Full size image To determine whether there is a loss of stem cell function with ageing and progeria, MDSPCs were isolated from old WT mice (2-yrs) as well as progeroid Ercc1 −/− (2–3-wks) and Ercc1 −/Δ (5-mths) mice and their proliferation and differentiation kinetics measured in vitro . As controls, MDSPCs were isolated from age-matched WT littermates of the progeroid mice and Xpa −/− (xeroderma pigmentosum complementation group A) mice (3-wks), which are defective in nucleotide excision repair of DNA like ERCC1-deficient mice, but do not age rapidly [37] . To measure proliferation of MDSPCs, an equivalent number of cells from each population were plated, and live-cell imaging (LCI) [38] was used to measure growth kinetics ( Fig. 1c ). Analysis of images captured from the different cell populations revealed that proliferation of MDSPCs isolated from the old WT, Ercc1 −/− and Ercc1 −/Δ mice, but not Xpa −/− mice, was significantly reduced relative to MDSPCs isolated from young WT mice (* P <0.05, Tukey's test). The average population-doubling time (PDT) was prolonged in MDSPCs isolated from old mice [18 hours (h)] and progeroid mice (20–27 h) compared with young WT mice (15 h) ( Fig. 1c ). In support of this, the division time (DT) of single cells tracked within the population, or analysed as isolated clones, was also prolonged for old WT-MDSPCs and ERCC1-deficient MDSPCs compared with young WT-MDSPCs ( Supplementary Table S1 ). These data demonstrate that the proliferation capacity of MDSPCs diminishes with age. To determine whether the capacity for myogenic differentiation is affected in old and progeroid MDSPCs, the cells were cultured to confluence and switched to differentiation medium (low serum). The young WT- and Xpa −/− MDSPCs fused to form multinucleated myotubes expressing fast myosin heavy chain (f-MyHC), a marker of terminal myogenic differentiation ( Fig. 1d ). In contrast, MDSPCs isolated from old WT and progeroid ERCC1-deficient mice formed significantly fewer and smaller myotubes indicating impaired differentiation ( Fig. 1d ; * P <0.001; Kruskal–Wallis ANOVA on ranks). The differentiation defect was confirmed by measuring the expression of myogenic differentiation markers MyHC, desmin, and myogenin ( Fig. 1e ). Myogenic differentiation of individual MDSPC clones from old and progeroid mice was also significantly reduced, compared with young WT mice ( Supplementary Fig. S1 ; * P <0.001, Kruskal–Wallis ANOVA on ranks). Similarly, osteogenic and chondrogenic differentiation of progeroid and old MDSPCs was attenuated compared with cells isolated from young WT mice ( Fig. 1b ). In contrast, the capacity for adipogenic differentiation was retained in aged MDSPCs. To determine whether the myogenic differentiation defect translated in vivo , MDSPCs isolated from progeroid mice were injected intramuscularly (IM) into mdx mice, a model of Duchenne's muscular dystrophy [39] . Indeed, cells derived from Ercc1 −/Δ mice had an impaired ability to regenerate muscle fibres in dystrophic muscle compared with young WT-MDSPCs ( Fig. 1f,g ; P <0.001, Mann–Whitney rank sum test). Cumulatively, these data provide evidence of a significant loss of stemness properties, including proliferation under clonogenic conditions, multipotential differentiation and tissue regeneration, in MDSPC populations isolated from old and progeroid mice. To rule out the possibility that the stem cell dysfunction was an artefact caused by extensive passaging of MDSPCs ex vivo , we measured the number of cells with stem/progenitor surface markers and capacity for myogenic differentiation at the earliest possible time point following isolation from skeletal muscle. Preplate 1 and 2 (pp1–2; Fig. 2a ), which constitute all cells directly isolated from skeletal muscle, were induced to differentiate within 24 h of isolation. f-MyHC positive myotube formation was impaired in cells isolated from the skeletal muscle of progeroid ERCC1-deficient mice compared with WT littermates ( Fig. 2b ). Similarly, expression of a second terminal myogenic differentiation marker, myogenin, was reduced in the ERCC1-deficient cells compared with WT controls ( Fig. 2c ). Twenty-four-hours post-isolation from skeletal muscle, those cells that remained nonadherent were stained for surface markers Sca-1, CD34 and CD45 and analysed by fluorescence-activated cell sorting (FACS) to quantify the mixed population of non-haematopoietic stem/progenitor cells in the muscle ( Fig. 2d ). Sca-1 is expressed on adult stem cells, a sub-population of myoblasts [40] , muscle-derived fibrogenic/adipogenic progenitors [41] , and a non-myogenic population of cells that emerge in muscle with ageing [42] . 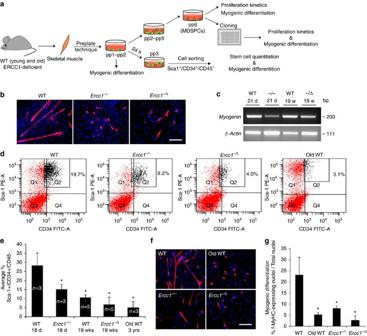Figure 2: Measuring the number of MDSPCs isolated from murine muscle and their myogenic potential. (a) A schematic diagram showing the early passage cells analysed in this figure and the method used to isolate various populations of MDSPCs (pp1–pp6). (b) Representative images of pp1–pp2 cells induced to undergo myogenic differentiation. Cells directly isolated from skeletal muscle of mice, using preplate technique (pp1–pp2), were incubated in fusion media to induce myogenic differentiation. Twenty-four hours post-isolation, adhering cells were trypsinized and plated at equal density and induced to undergo myogenic differentiation over 2–3 days. Cells from 2–3 independent populations of each genotype were immunostained for the terminal myogenic differentiation marker, f-MyHC (red). Scale bar=100 μm. (c) rtPCR to measure the expression of the myogenic differentiation marker, myogenin in pp1–pp2 cells, induced to undergo myogenic differentiation. (d) Quantification of Sca-1+/CD34+/CD45−cells in young WT-, old WT-, and progeroid- (Ercc1−/−,Ercc1−/Δ) murine skeletal muscle. Twenty-four hours after isolation from muscle, the cells that did not adhere in preplate 1 and 2 (that is, pp3) were analysed for stem/progenitor cell markers by FACS. The number in the upper right quadrants indicates the percent of Sca-1+/CD34+/CD45−cells isolated from 3–5 mice of each genotype/age. (e) Graph indicating the average fraction of Sca-1+/CD34+/CD45−cells normalized to the weight of the cell pellet of pp3 cell populations. Error bars indicate ±s.d. *P<0.05, Tukey's test, relative to young WT cells. (f) Representative images of Sca-1+/CD34+/CD45−-sorted cells plated at equal density and induced to undergo myogenic differentiation. The cells were stained for the terminal myogenic marker, f-MyHC (red). Scale bar=100 μm. (g) Quantification of myogenic differentiation of Sca-1+/CD34+/CD45−cells isolated from the skeletal muscle of mice of various genotypes/ages measured as the percent of cells (DAPI, blue) expressing f-MyHC (red). Error bars indicate ±s.d. for cell populations isolated from 2–3 animals per genotype *P<0.001, Kruskal–Wallis ANOVA on ranks relative to young WT cells. Figure 2: Measuring the number of MDSPCs isolated from murine muscle and their myogenic potential. ( a ) A schematic diagram showing the early passage cells analysed in this figure and the method used to isolate various populations of MDSPCs (pp1–pp6). ( b ) Representative images of pp1–pp2 cells induced to undergo myogenic differentiation. Cells directly isolated from skeletal muscle of mice, using preplate technique (pp1–pp2), were incubated in fusion media to induce myogenic differentiation. Twenty-four hours post-isolation, adhering cells were trypsinized and plated at equal density and induced to undergo myogenic differentiation over 2–3 days. Cells from 2–3 independent populations of each genotype were immunostained for the terminal myogenic differentiation marker, f-MyHC (red). Scale bar=100 μm. ( c ) rtPCR to measure the expression of the myogenic differentiation marker, myogenin in pp1–pp2 cells, induced to undergo myogenic differentiation. ( d ) Quantification of Sca-1 + /CD34 + /CD45 − cells in young WT-, old WT-, and progeroid- ( Ercc1 −/− , Ercc1 −/Δ ) murine skeletal muscle. Twenty-four hours after isolation from muscle, the cells that did not adhere in preplate 1 and 2 (that is, pp3) were analysed for stem/progenitor cell markers by FACS. The number in the upper right quadrants indicates the percent of Sca-1 + /CD34 + /CD45 − cells isolated from 3–5 mice of each genotype/age. ( e ) Graph indicating the average fraction of Sca-1 + /CD34 + /CD45 − cells normalized to the weight of the cell pellet of pp3 cell populations. Error bars indicate ±s.d. * P <0.05, Tukey's test, relative to young WT cells. ( f ) Representative images of Sca-1 + /CD34 + /CD45 − -sorted cells plated at equal density and induced to undergo myogenic differentiation. The cells were stained for the terminal myogenic marker, f-MyHC (red). Scale bar=100 μm. ( g ) Quantification of myogenic differentiation of Sca-1 + /CD34 + /CD45 − cells isolated from the skeletal muscle of mice of various genotypes/ages measured as the percent of cells (DAPI, blue) expressing f-MyHC (red). Error bars indicate ±s.d. for cell populations isolated from 2–3 animals per genotype * P <0.001, Kruskal–Wallis ANOVA on ranks relative to young WT cells. Full size image In young WT mice, ∼ 20% of the cells were Sca-1 + /CD34 + /CD45 − . In contrast, <10% of the cells isolated from old or progeroid skeletal muscle were Sca-1 + /CD34 + /CD45 − . Averaging data from 3–5 populations of each genotype revealed a significant depletion of this population of cells as animal age ( Fig. 2e ; * P <0.05; Tukey's test). Next, we plated an equivalent number of these sorted cells to directly compare the myogenic differentiation capacity between Sca-1 + /CD34 + /CD45 − cells from the different genotypes and ages of mice. Myogenic differentiation was significantly impaired in cells isolated from old or progeroid mice compared with young WT mice ( Fig. 2f,g ; * P <0.001; Kruskal–Wallis ANOVA on ranks). These data demonstrate that there is a loss of MDSPC cell number as well as capacity for myogenic differentiation with ageing. To determine whether there is a difference in the function of muscle stem cells between aged and young organisms in vivo , we examined muscle regeneration utilizing a well-established cardiotoxin injury-induced model ( Supplementary Methods ) [43] . The total area of muscle regeneration, as defined by centronucleated fibres, did not significantly differ between young WT, old WT, and progeroid mice ( Supplementary Table S2 ). However, there was a dramatic difference in the average cross-sectional area of the regenerated myofibres in old and progeroid mice compared with young adult mice ( Fig. 3a ). More than 50% of the centronucleated, dystrophin-positive myofibres in old and progeroid mice had an area of ≤ 500 μm 2 ( Fig. 3b ). In contrast, >60% of the myofibres in young WT mice had an area of >1,000 μm 2 , indicative of significantly more mature regenerated myofibres ( P <0.001; Kruskal–Wallis ANOVA on ranks). In addition, Masson's Trichrome stain revealed increased fibrosis in muscle of old and progeroid mice in comparison to young WT mice following injury ( Fig. 3c,d ; * P <0.05; Tukey's test). These data demonstrate that muscle regeneration is delayed and impaired in aged organisms. Collectively, the data in Figures 2 and 3 support the conclusion that aged organisms have a muscle stem/progenitor cell defect. 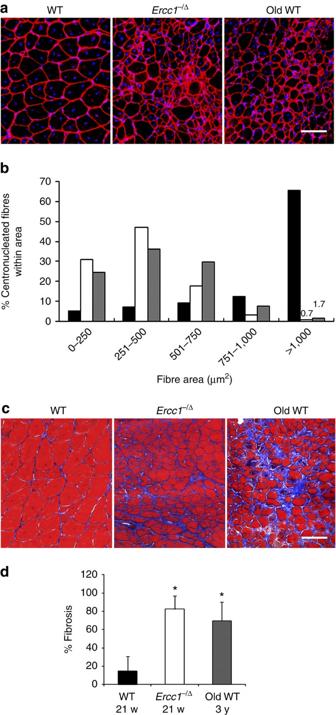Figure 3: Measuring muscle regeneration after injury in old and progeroid mice. To measure muscle stem/progenitor cell functionin vivo, cardiotoxin was injected directly into the gastrocnemius muscle of old WT (3-yr-old;n=3), adult WT (18–21-wk-old;n=5), and progeroidErcc1−/Δ(21-wk-old;n=2 plus 8-wk-old;n=3) mice to induce muscle injury. Two wks later, tissues were collected and stained for dystrophin (red) and nuclei (DAPI). (a) Representative images of damaged muscle sections. Scale bar=100 μm. (b) Quantification of the cross-sectional area of regenerating myofibres after muscle injury of adult WT mice (black bars), progeroidErcc1−/Δlittermates (white bars) and old WT mice (grey bars). The area of >1,000 myofibres was measured per group of mice. The distribution of fibre size is indicated on thex-axis, representing increasingly more mature fibres with increased size. The fraction of regenerating, centronucleated myofibres of each size range is plotted. (P<0.001, Kruskal–Wallis ANOVA on ranks at 0–250, 251–500, and >1,000). (c) Trichrome staining of sections from the same damaged muscles to reveal areas of fibrosis (blue). Shown are representative images from 1 of 2–3 mice of each genotype analysed. (d) Histogram indicating the area of fibrotic scarring following cardiotoxin injection. Plotted is the average fraction (n=2–3 animals per genotype/age) of the area examined that is fibrotic in percent ±s.d. *P<0.05, Tukey's test, relative to young WT. Scale bar=100 μm. Figure 3: Measuring muscle regeneration after injury in old and progeroid mice. To measure muscle stem/progenitor cell function in vivo , cardiotoxin was injected directly into the gastrocnemius muscle of old WT (3-yr-old; n =3), adult WT (18–21-wk-old; n =5), and progeroid Ercc1 −/Δ (21-wk-old; n =2 plus 8-wk-old; n =3) mice to induce muscle injury. Two wks later, tissues were collected and stained for dystrophin (red) and nuclei (DAPI). ( a ) Representative images of damaged muscle sections. Scale bar=100 μm. ( b ) Quantification of the cross-sectional area of regenerating myofibres after muscle injury of adult WT mice (black bars), progeroid Ercc1 −/Δ littermates (white bars) and old WT mice (grey bars). The area of >1,000 myofibres was measured per group of mice. The distribution of fibre size is indicated on the x -axis, representing increasingly more mature fibres with increased size. The fraction of regenerating, centronucleated myofibres of each size range is plotted. ( P <0.001, Kruskal–Wallis ANOVA on ranks at 0–250, 251–500, and >1,000). ( c ) Trichrome staining of sections from the same damaged muscles to reveal areas of fibrosis (blue). Shown are representative images from 1 of 2–3 mice of each genotype analysed. ( d ) Histogram indicating the area of fibrotic scarring following cardiotoxin injection. Plotted is the average fraction ( n =2–3 animals per genotype/age) of the area examined that is fibrotic in percent ±s.d. * P <0.05, Tukey's test, relative to young WT. Scale bar=100 μm. Full size image Treating with young WT-MDSPCs extends life and healthspan To determine whether the loss of functional MDSPCs contributes to ageing-related degenerative changes, we asked whether transplantation of young WT-MDSPCs affects either the healthspan or lifespan of progeroid mice. Littermate pairs of Ercc1 −/− mice were injected intraperitoneally (IP) with 2–4×10 5 young WT-, progeroid-, or old WT-MDSPCs per gram body weight or PBS at 17 days of age, and lifespan was measured (summarized in Supplementary Table S3 ). Ercc1 −/− mice injected with young WT-MDSPCs showed pronounced weight gain and a significantly extended lifespan compared with sibling mutant animals injected with vehicle only ( Fig. 4a ; * P <0.05, Dunn's test). In an identical experiment, early passage primary mouse embryonic fibroblasts (MEFs) did not affect the growth or lifespan of Ercc1 −/− mice ( Fig. 4a ). Similarly, MDSPCs isolated from old WT or progeroid Ercc1 −/− mice did not have a significant impact on lifespan. 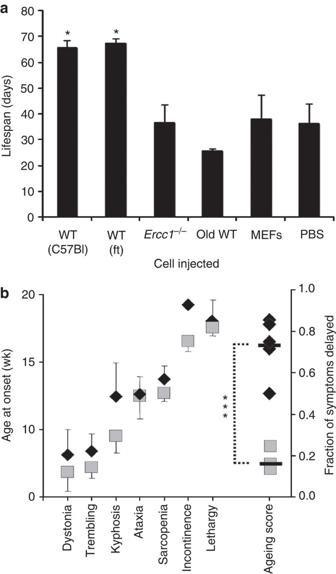Figure 4: Measuring the impact of MDSPC transplantation on the lifespan and healthspan of progeroid mice. (a) 2–4×105MDSPCs per gram body weight were injected into the peritoneal cavity of 17-day-oldErcc1−/−mice and lifespan measured. The median lifespan ofErcc1−/−mice is 21 days; the maximum is 28 days29. The lifespan ofErcc1−/−mice injected with two independent MDSPC populations isolated from young WT mice were compared withErcc1−/−mice injected with vehicle only (PBS), an equivalent number of WT MEFs, or MDSPCs isolated from old WT or progeroidErcc1−/−mice. Reported is the average lifespan from 4–10 mice injected per treatment group. Error bars indicate s.e.m. *P<0.05, Dunn's test comparing the WT groups with all other treatment groups. A summary of the cell lines injected and number of animals transplanted can be found inSupplementary Table S3. (b) 2–4 ×105MDSPCs per gram body weight were injected into the peritoneal cavity of 7-wk-oldErcc1−/Δmice and again at 13 wks of age. The age at onset of the characteristic, spontaneous, ageing-related symptoms seen inErcc1−/Δmice was measured (MDSPC-treated mice, black diamonds) and compared with mice injected with vehicle only (PBS; grey squares). Reported is the average age at onset of each progeroid symptom in wks ±s.d. (n=8 mice per treatment group). The ageing score is calculated as the fraction of symptoms that were delayed in a singleErcc1−/Δmice injected with young WT-MDSPCs compared with an age- and sex-matched mouse (usually a littermate) injected with PBS (Supplementary Methods). The black bars denote the average ageing score for each group (***P<0.0008, Student'st-test). Figure 4: Measuring the impact of MDSPC transplantation on the lifespan and healthspan of progeroid mice. ( a ) 2–4×10 5 MDSPCs per gram body weight were injected into the peritoneal cavity of 17-day-old Ercc1 −/− mice and lifespan measured. The median lifespan of Ercc1 −/− mice is 21 days; the maximum is 28 days [29] . The lifespan of Ercc1 −/− mice injected with two independent MDSPC populations isolated from young WT mice were compared with Ercc1 −/− mice injected with vehicle only (PBS), an equivalent number of WT MEFs, or MDSPCs isolated from old WT or progeroid Ercc1 −/− mice. Reported is the average lifespan from 4–10 mice injected per treatment group. Error bars indicate s.e.m. * P <0.05, Dunn's test comparing the WT groups with all other treatment groups. A summary of the cell lines injected and number of animals transplanted can be found in Supplementary Table S3 . ( b ) 2–4 ×10 5 MDSPCs per gram body weight were injected into the peritoneal cavity of 7-wk-old Ercc1 −/Δ mice and again at 13 wks of age. The age at onset of the characteristic, spontaneous, ageing-related symptoms seen in Ercc1 −/Δ mice was measured (MDSPC-treated mice, black diamonds) and compared with mice injected with vehicle only (PBS; grey squares). Reported is the average age at onset of each progeroid symptom in wks ±s.d. ( n =8 mice per treatment group). The ageing score is calculated as the fraction of symptoms that were delayed in a single Ercc1 −/Δ mice injected with young WT-MDSPCs compared with an age- and sex-matched mouse (usually a littermate) injected with PBS ( Supplementary Methods ). The black bars denote the average ageing score for each group (*** P <0.0008, Student's t -test). Full size image The young WT-MDSPCs were also injected IP into Ercc1 −/Δ mice at 6–7 wks of age and again 6 wks later. The age at onset of characteristic progeroid symptoms was measured biweekly, including dystonia, trembling, kyphosis, ataxia, muscle wasting, loss of vision, urinary incontinence and decreased spontaneous activity. The results were compared with littermate Ercc1 −/Δ mice treated with vehicle only in a pairwise fashion. The investigators were blinded to the treatment arm. The ageing score, representing the fraction of symptoms that were delayed in mutant mice treated with MDSPCs compared with a mutant littermate treated with PBS, revealed a highly significant difference between treatment groups ( Fig. 4b ; *** P <0.0008; Student's t -test). These data provide evidence that loss of stem cell function has a direct causal role in ageing-related degeneration. Young WT-MDSPCs engraft after transplantation To address the question of how MDSPCs could extend healthspan and lifespan, we asked whether the donor cells engrafted in host tissues. Young WT-MDSPCs, transduced with a retroviral vector containing LacZ with a nuclear localization sequence ( nLacZ ), were injected IP into Ercc1 −/− mice ( n =8). Fourteen tissues were analysed ( Supplementary Table S4 ) for the presence of donor cells. LacZ + cells were detected in the parenchyma of the liver and kidney, as well as connective tissues associated with pancreas and spleen of all mice analysed ( Fig. 5 ). Similar results were obtained in animals euthanized from 1 to 9 wks post-injection. LacZ + cells were also detected in lung, oesophagus, thymus, bladder/ureter, spinal cord, and bone marrow of at least one mouse ( Fig. 5 ; Supplementary Fig. S2 ). Importantly, donor cells were not detected in the heart, brain, skeletal muscles, and lymph nodes of any mice. The extent of donor cell engraftment and expansion is limited, indicating that the beneficial effects of MDSPCs is not due to tissue reconstitution by donor cells as is seen with haematopoietic stem cells in bone marrow transplant. 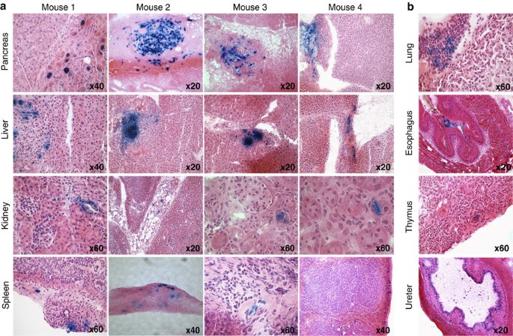Figure 5: Determination of the site for donor cell engraftment of young WT-MDSPCs. 2–4 ×105young WT-MDSPCs expressing nuclearLacZper gram body weight were injected IP intoErcc1−/−mice to determine the sites of engraftment. Mice were injected at 12 days of age and euthanized 8–9 days later (n=4) or injected at 17–19 days of age and tissues collected at the end of their lifespan (4–9-wks of age;n=4). Fourteen organs/tissues were isolated, sectioned and stained with X-gal to identify donor cells (Supplementary Table S4). (a) Donor cells (LacZ+ stained blue) were detected in the pancreas, liver, spleen, and kidney of all host animals. Shown are representative images from four mice illustrating the site and extent of engraftment of donor cells. (b) Donor cells were detected in the lung, esophagus, thymus and ureter of at least one mouse. Shown are images at multiple levels of magnification from tissue sections of one mouse per organ to illustrate the site and extent of engraftment. The level of magnification is indicated for each tissue section image. Figure 5: Determination of the site for donor cell engraftment of young WT-MDSPCs. 2–4 ×10 5 young WT-MDSPCs expressing nuclear LacZ per gram body weight were injected IP into Ercc1 −/− mice to determine the sites of engraftment. Mice were injected at 12 days of age and euthanized 8–9 days later ( n =4) or injected at 17–19 days of age and tissues collected at the end of their lifespan (4–9-wks of age; n =4). Fourteen organs/tissues were isolated, sectioned and stained with X-gal to identify donor cells ( Supplementary Table S4 ). ( a ) Donor cells ( LacZ + stained blue) were detected in the pancreas, liver, spleen, and kidney of all host animals. Shown are representative images from four mice illustrating the site and extent of engraftment of donor cells. ( b ) Donor cells were detected in the lung, esophagus, thymus and ureter of at least one mouse. Shown are images at multiple levels of magnification from tissue sections of one mouse per organ to illustrate the site and extent of engraftment. The level of magnification is indicated for each tissue section image. Full size image Young WT-MDSPCs restore the function of aged MDSPCs In a progeria model ( Ercc1 −/− mice), young WT-MDSPCs had a therapeutic effect. However, the duration of the experiment (<3 wks) and the limited extent of engraftment of IP-injected MDSPCs, as far as we could detect, made it unlikely that this positive effect was a result of substantial MDSPC engraftment, proliferation, differentiation and tissue regeneration. Thus, we next asked whether young WT-MDSPCs confer their therapeutic effects through a paracrine mechanism, requiring secreted factors. MDSPCs isolated from 14-day-old progeroid Ercc1 −/− mice were co-cultured with the young WT-MDSPCs, using a transwell system ( Fig. 6a ). The proliferation of Ercc1 −/− MDSPCs was measured for 72 h while the cells were exposed to proliferation media from young WT-MDSPCs. Subsequently, the Ercc1 −/− MDSPCs were switched to low-serum media to measure myogenic differentiation. The proliferation defect of Ercc1 −/− MDSPCs was significantly improved by co-culture of the cells with young WT-MDSPCs ( Fig. 6b ; * P <0.001, Mann–Whitney rank sum test). In addition, myogenic differentiation of Ercc1 −/− MDSPCs was improved after co-culture with young WT-MDSPCs ( Fig. 6c ). Likewise, impaired differentiation of old WT-MDSPCs was rescued by conditioned media from young WT-MDSPCs. To quantify the improvement, MDSPCs from progeroid Ercc1 −/− or old WT mice were grown in the presence of conditioned media from young WT-MDSPCs, then collected for immunodetection of the terminal myogenic differentiation marker f-MyHC ( Fig. 6d ). f-MyHC expression was dramatically increased (2.5–9×) if the cells were grown in the presence of media from young WT-MDSPCs compared with differentiation media alone. Thus young WT-MDSPCs were able to rescue, at least in part, the function (proliferation and differentiation) of MDSPCs isolated from progeroid and old mice via secreted factors. 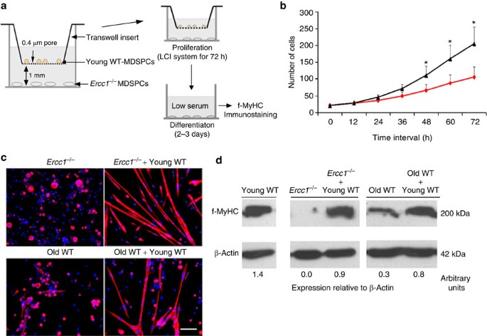Figure 6: Measurement of proliferation and myogenic differentiation of MDSPCs co-cultured with young WT-MDSPCs. (a) A schematic diagram of the co-culture system used to evaluate the effect of young functional MDSPCs on dysfunctional MDSPCs isolated from progeroid or old WT mice.Ercc1−/−MDSPCs were plated in the lower compartment of the transwell system in proliferation media. WT-MDSPCs were seeded onto the upper transwell membrane inserts, at the same density, and in the same media. These co-cultures were placed in the LCI system for 72 h to acquire time-lapsed images to measure proliferation of the MDSPCs. As a control, each plate contained wells ofErcc1−/−MDSPCs without transwell membrane inserts. (b) Plotted is the average cell number at each time point calculated from the analysis of three independent populations ofErcc1−/−MDSPCs co-cultured with young WT-MDSPCs (black line), or without (red line) ±s.d. *P<0.001, Mann–Whitney rank sum test. (c) The transwell inserts were removed after 72 h and the proliferation media was switched to differentiation media. After 2–3 days, myogenic differentiation ofErcc1−/−and old WT-MDSPC was tested by immunostaining the cells for f-MyHC (red). Shown are representative images. The nuclear counterstain is DAPI (blue). Scale bar=100 μm. (d) Quantification of myogenic differentiation of old WT-MDSPCs after growth in media conditioned from young WT-MDSPCs. Young WT-MDSPCs were cultured for 2 days in proliferation media in collagen-coated flasks, then treated with differentiation media for 3 days. The supernatant from these cultures was collected for use as conditioned media. MDSPCs from 21-day-old progeroidErcc1−/−mice and 2-yr-old WT mice were grown in the presence of this conditioned media or unconditioned differentiation media to determine the impact on myogenic differentiation as measured by immunoblot detection of f-MyHC. Densitometric quantification of f-MyHC corrected for β-Actin is indicated below each lane. Figure 6: Measurement of proliferation and myogenic differentiation of MDSPCs co-cultured with young WT-MDSPCs. ( a ) A schematic diagram of the co-culture system used to evaluate the effect of young functional MDSPCs on dysfunctional MDSPCs isolated from progeroid or old WT mice. Ercc1 −/− MDSPCs were plated in the lower compartment of the transwell system in proliferation media. WT-MDSPCs were seeded onto the upper transwell membrane inserts, at the same density, and in the same media. These co-cultures were placed in the LCI system for 72 h to acquire time-lapsed images to measure proliferation of the MDSPCs. As a control, each plate contained wells of Ercc1 −/− MDSPCs without transwell membrane inserts. ( b ) Plotted is the average cell number at each time point calculated from the analysis of three independent populations of Ercc1 −/− MDSPCs co-cultured with young WT-MDSPCs (black line), or without (red line) ±s.d. * P <0.001, Mann–Whitney rank sum test. ( c ) The transwell inserts were removed after 72 h and the proliferation media was switched to differentiation media. After 2–3 days, myogenic differentiation of Ercc1 −/− and old WT-MDSPC was tested by immunostaining the cells for f-MyHC (red). Shown are representative images. The nuclear counterstain is DAPI (blue). Scale bar=100 μm. ( d ) Quantification of myogenic differentiation of old WT-MDSPCs after growth in media conditioned from young WT-MDSPCs. Young WT-MDSPCs were cultured for 2 days in proliferation media in collagen-coated flasks, then treated with differentiation media for 3 days. The supernatant from these cultures was collected for use as conditioned media. MDSPCs from 21-day-old progeroid Ercc1 −/− mice and 2-yr-old WT mice were grown in the presence of this conditioned media or unconditioned differentiation media to determine the impact on myogenic differentiation as measured by immunoblot detection of f-MyHC. Densitometric quantification of f-MyHC corrected for β-Actin is indicated below each lane. Full size image MDSPCs promote neovascularization and tissue regeneration To determine whether secreted factors were indeed important for the therapeutic effect of MDSPCs, we asked whether there was evidence of improved histopathology in tissues of treated ERCC1-deficient mice in which transplanted MDSPCs were not detected, in particular, skeletal muscle and brain. We previously demonstrated that the regenerative potential of MDSPCs transplanted into skeletal muscle, heart and bone correlates with their ability to induce angiogenesis [21] , [24] , [25] , [35] , [44] . Thus, we asked whether IP injection of young WT-MDSPCs had an effect on the vasculature of the brain, as well as muscle fibre size. Muscle sections were stained for dystrophin to highlight muscle fibre perimeter and CD31 to identify endothelial cells within microvessels ( Fig. 7a ). For each image, the total number of muscle fibres and CD31+ cells were quantified, and the ratio (# of CD31+ cells/# of muscle fibres) determined. Muscles of 15-day-old Ercc1 −/− mice had significantly reduced numbers of CD31+ cells at the periphery of muscle fibres compared with WT littermates ( Fig. 7b ; 0.56 CD31+ cells per fibre versus 1.25 for WT mice; * P <0.001, Student's t -test). The average muscle-fibre size was also significantly reduced in the Ercc1 −/− mice (324 μm 2 ) compared with WT littermates ( Fig. 7b ; 734 μm 2 , * P =0.002, Mann–Whitney rank sum test). 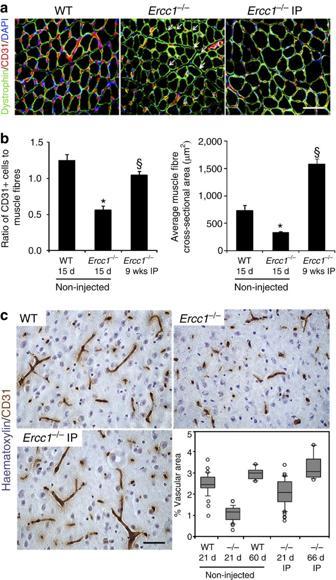Figure 7: Host muscle fibre size and tissue vascularization following intraperitoneal transplantation of young WT-MDSPCs. (a) Representative sections from the gastrocnemius muscle of 15-day-old WT andErcc1−/−mice, as well asErcc1−/−mice transplanted with young WT-MDSPCs at 17 days of age and allowed to live their full lifespan (Ercc1−/−IP), immunostained for dystrophin (green), CD31 (red), and DAPI (blue). Arrows indicate myofibres lacking adjacent CD31+ cells (microvasculature). Scale bars=100 μm. (b) Quantification of microvasculature and myofibre size in these mice. Images from 4–8 sections and 500–1,000 fibres from 3 animals per group were analysed. Reported are the ratio of CD31+ cells to dystrophin-positive muscle fibres (left) and the average muscle fibre size (cross-sectional area; right). Error bars indicate s.e.m. *P<0.001, Student'st-test comparing theErcc1−/−mice with WT mice and§P<0.05, Tukey's test comparing untreated and treatedErcc1−/−mice; for myofibre size *P=0.002, Mann–Whitney rank sum test comparing theErcc1−/−mice with WT mice and§P<0.05, Dunn's Method comparing untreated and treatedErcc1−/−mice. (c) Representative images from sections of the cerebral cortex of 21-day-old WT andErcc1−/−mice, andErcc1−/−mice transplanted with young WT-MDSPCs. Tissue sections were stained for CD31 to detect the microvasculature. The percent of the tissue area representing vasculature was quantified using bright field images and Northern Eclipse software. Each circle plotted represents an individual mouse. The horizontal bar is the median (50th percentile) area. The box represents the 25th–75th percentile, and the error bars represent the 10th–90th percentile. Figure 7: Host muscle fibre size and tissue vascularization following intraperitoneal transplantation of young WT-MDSPCs. ( a ) Representative sections from the gastrocnemius muscle of 15-day-old WT and Ercc1 −/− mice, as well as Ercc1 −/− mice transplanted with young WT-MDSPCs at 17 days of age and allowed to live their full lifespan ( Ercc1 −/− IP), immunostained for dystrophin (green), CD31 (red), and DAPI (blue). Arrows indicate myofibres lacking adjacent CD31+ cells (microvasculature). Scale bars=100 μm. ( b ) Quantification of microvasculature and myofibre size in these mice. Images from 4–8 sections and 500–1,000 fibres from 3 animals per group were analysed. Reported are the ratio of CD31+ cells to dystrophin-positive muscle fibres (left) and the average muscle fibre size (cross-sectional area; right). Error bars indicate s.e.m. * P <0.001, Student's t -test comparing the Ercc1 −/− mice with WT mice and § P <0.05, Tukey's test comparing untreated and treated Ercc1 −/− mice; for myofibre size * P =0.002, Mann–Whitney rank sum test comparing the Ercc1 −/− mice with WT mice and § P <0.05, Dunn's Method comparing untreated and treated Ercc1 −/− mice. ( c ) Representative images from sections of the cerebral cortex of 21-day-old WT and Ercc1 −/− mice, and Ercc1 −/− mice transplanted with young WT-MDSPCs. Tissue sections were stained for CD31 to detect the microvasculature. The percent of the tissue area representing vasculature was quantified using bright field images and Northern Eclipse software. Each circle plotted represents an individual mouse. The horizontal bar is the median (50th percentile) area. The box represents the 25th–75th percentile, and the error bars represent the 10th–90th percentile. Full size image IP injection of young WT-MDSPCs into Ercc1 −/− mice led to a significant increase in the number of CD31+ cells 9 wks post-injection compared with untreated Ercc1 −/− mice that only live 3–4 wks ( Fig. 7b ; 1.05 CD31+ vessels/fibre; § P <0.05, Tukey's test). Similarly, muscle-fibre size significantly increased ( Fig. 7b ; 1,580 μm 2 cross-sectional area; § P <0.05, Dunn's test). It is impossible to directly compare the fibre size between Ercc1 −/− mice transplanted with young WT-MDSPCs to untreated mutant animals of the same age because the latter don't live to 9 wks of age ( Fig. 4a ). Nevertheless, muscle regeneration and growth was evident in Ercc1 −/− mice treated with MDSPCs. Progeroid Ercc1 −/− mice show reduced vascularization in the brain compared with WT littermates at 3 wks of age ( Fig. 7c ; Supplementary Fig. S3 ). Although donor cells were not detected in the brain of Ercc1 −/− mice, cell transplantation significantly improved neovascularization in the brain of these progeroid mice. In 3-wk-old Ercc1 −/− mice, the median area of cerebral cortex occupied by vasculature was 1.2%. In Ercc1 −/− mice injected with MDSPCs, vascularization increased approximately to the levels in 3-wk-old WT mice (2.2 versus 2.5%, respectively) and the improvement was sustained. Ercc1 −/− mice treated with MDSPCs that survived to 9 wks of age, had a vascular area indistinguishable from age-matched WT mice (3.2 versus 3.1%, P <0.05, Dunn's test). These data demonstrate that there is improvement in the histopathology of several tissues in which donor cell engraftment was not detected, suggesting that MDSPCs exert their therapeutic effect through secreted factors. Using IM injection of nLacZ -labelled MDSPCs to localize donor-cell engraftment, we analysed host muscle for presence of LacZ + myofibres and endothelial cells ( Fig. 8 ). Like IP, IM administration of young WT-MDSPCs into Ercc1 −/− mice ( Fig. 8a , n =3 mice per group) led to a significant increase in the number of CD31+ cells ( Fig. 8b ; 1.06 CD31+ vessels per fibre; § P <0.05, Tukey's test) compared with the non-injected Ercc1 −/− mice (0.56 CD31+ vessels/fibre). The muscle-fibre cross-sectional area was also significantly increased ( Fig. 8b ; 522 versus 324 μm 2 , § P <0.05, Dunn's test). At the site of injection, numerous myofibres with central or peripheral LacZ + nuclei were identified, demonstrating that transplanted MDSPCs have the capacity to integrate into regenerated muscle fibres ( Fig. 8c ). In addition, analysis of sections of the gastrocnemius distant from the injection site revealed a shift in the distribution of myofibre size towards larger regenerating fibres compared with contralateral non-injected muscle ( Fig. 8d ; P <0.001, Mann–Whitney rank sum test at 151–300 and 301–450). This suggests that IM injection of MDSPCs also affected host myofibres through a paracrine mechanism, requiring secreted factors. Sections were also stained with X-gal and for CD31 to determine whether donor cells co-localize with CD31+ cells ( Fig. 8e ). Background staining in Ercc1 −/− mice was extensive, compared with mdx /SCID mice, likely due to interstitial fibrosis. In both cases, there was a lack of co-localization of LacZ and CD31 staining. These data are consistent with our previous findings [25] , [45] and the conclusion that transplanted MDSPCs do not directly contribute to blood vessels and thus likely drive host angiogenesis through secreted factors. 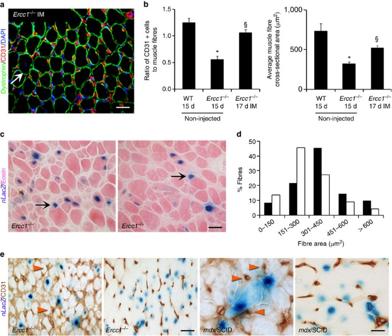Figure 8: Measurement of host muscle fibre size and tissue vascularization after intramuscular transplantation with young WT-MDSPCs. (a) The gastrocnemius muscle of 12-day-oldErcc1−/−mice (n=3 mice) was injected with young WT-MDSPCs. Tissues were isolated 5 days later (17 d) and sections were immunostained for dystrophin (green), CD31 (red), and DAPI (blue) and compared with untreated 15-day-old WT andErcc1−/−mice (fromFig. 7). The white arrow denotes a centronucleated fibre. Scale bar=100 μm. (b) Quantification of microvasculature and myofibre size in transplanted and untreated mice. Images from 4–8 sections from 3 animals per group were analysed. Reported is the ratio of CD31+cells to dystrophin-positive muscle fibres (left),§P<0.05 between untreated and treatedErcc1−/−mice, Tukey's test. On the right is the average muscle fibre size (cross-sectional area),§P<0.05 between untreated and treatedErcc1−/−mice, Dunn's test. Error bars indicate s.e.m. (c) Seventeen day-old progeroidErcc1−/−mice (n=10) were injected IM with WT-MDSPCs expressing nuclearLacZto determine whether donor cells integrate into muscle fibres and contribute to blood vessels. Five days later, the mice were euthanized and the gastrocnemius muscles were isolated for analysis. Muscle sections at the injection site were stained with X-gal, to detect donor cells, and eosin. Scale bar=50 μm. (d) Histogram of the cross-sectional area distribution of myofibres in the treated gastrocnemius muscles (black bars) compared the contralateral non-injected muscle (white bars). Data were collected from 6,000 fibres from multiple sections of four mice per group. The distribution of fibre size is indicated on thex-axis, representing increasingly more mature fibres with increased size (P<0.001, Mann–Whitney rank sum test at 151–300 and 301–450). (e) Sections from the injected muscles stained for CD31 to identify blood vessels (dark brown) and X-gal to identify donor cells (blue). Red arrowheads indicate CD31+ capillary structures. Sections from dystrophic (mdx/SCID) mice treated the same way are included as a positive control (right panels). Scale bars=50 μm. Figure 8: Measurement of host muscle fibre size and tissue vascularization after intramuscular transplantation with young WT-MDSPCs. ( a ) The gastrocnemius muscle of 12-day-old Ercc1 −/− mice ( n =3 mice) was injected with young WT-MDSPCs. Tissues were isolated 5 days later (17 d) and sections were immunostained for dystrophin (green), CD31 (red), and DAPI (blue) and compared with untreated 15-day-old WT and Ercc1 −/− mice (from Fig. 7 ). The white arrow denotes a centronucleated fibre. Scale bar=100 μm. ( b ) Quantification of microvasculature and myofibre size in transplanted and untreated mice. Images from 4–8 sections from 3 animals per group were analysed. Reported is the ratio of CD31 + cells to dystrophin-positive muscle fibres (left), § P <0.05 between untreated and treated Ercc1 −/− mice, Tukey's test. On the right is the average muscle fibre size (cross-sectional area), § P <0.05 between untreated and treated Ercc1 −/− mice, Dunn's test. Error bars indicate s.e.m. ( c ) Seventeen day-old progeroid Ercc1 −/− mice ( n =10) were injected IM with WT-MDSPCs expressing nuclear LacZ to determine whether donor cells integrate into muscle fibres and contribute to blood vessels. Five days later, the mice were euthanized and the gastrocnemius muscles were isolated for analysis. Muscle sections at the injection site were stained with X-gal, to detect donor cells, and eosin. Scale bar=50 μm. ( d ) Histogram of the cross-sectional area distribution of myofibres in the treated gastrocnemius muscles (black bars) compared the contralateral non-injected muscle (white bars). Data were collected from 6,000 fibres from multiple sections of four mice per group. The distribution of fibre size is indicated on the x -axis, representing increasingly more mature fibres with increased size ( P <0.001, Mann–Whitney rank sum test at 151–300 and 301–450). ( e ) Sections from the injected muscles stained for CD31 to identify blood vessels (dark brown) and X-gal to identify donor cells (blue). Red arrowheads indicate CD31+ capillary structures. Sections from dystrophic ( mdx /SCID) mice treated the same way are included as a positive control (right panels). Scale bars=50 μm. Full size image MDSPCs are stem/progenitor cells isolated from skeletal muscle, a tissue that universally declines in mass and function with ageing [20] . This cell population cannot be discriminated from less multipotent progenitors strictly based on surface markers, and thus are difficult to quantify. Nevertheless, MDSPCs were isolated from old WT mice and mice with accelerated ageing, using a well-established preplate technique [21] , [22] . In both cases, cell proliferation and multilineage differentiation is significantly impaired relative to MDSPCs isolated from young WT mice ( Fig. 1 ). Furthermore, fewer cells expressing stem/progenitor cell markers are isolated from skeletal muscles of aged and progeroid mice ( Fig. 2 ). Finally, muscle from aged and progeroid mice has significantly reduced regenerative capacity following injury ( Fig. 3 ; Supplementary Table S2 ), consistent with previous reports [11] . These data establish that the function of MDSPCs is compromised with ageing, similar to neuronal, mesenchymal, haematopoietic, satellite, and adipose stem cells [4] , [15] , [17] , [46] , [47] , [48] . The similarity of deficits in MDSPCs from old WT and progeroid mice extends the commonalities between accelerated ageing caused by a defect in DNA repair and natural ageing. Similar parallels were found between Hutchinson-Gilford progeria syndrome and ageing in the MSC compartment [49] . Numerous studies provide evidence that the number and/or function of diverse adult stem cell populations decline with ageing [4] , [6] , [7] , [15] , [47] , [50] , [51] . However, these are largely correlative studies that do not discriminate whether changes in the stem cell compartment have a causative role in ageing or are merely a consequence of ageing. Genetic studies revealed proteins and pathways essential for the maintenance of stem cell function. Mutation of these genes leads to foreshortened lifespan and early onset of some ageing-related pathologies. For example, mice deficient in the polycomb protein BMI-1 have a short lifespan [52] , along with defects in self-renewal of HSCs, leading to adult stem cell depletion [53] . Similarly, mice deficient in HMGA2 show reduced stem cell numbers and function (self-renewal) throughout the central and peripheral nervous systems [54] . Finally, HSC function and regenerative capacity are significantly diminished in mice harbouring mutations in diverse DNA repair genes or telomerase ( Lig4 Y288C , Ku80 −/− , Xpd TTD , and mTR −/− ) indicating that genome and telomere maintenance are crucial for stem cell function [55] , [56] . However, there is no evidence that loss of stem cell function is directly responsible for decreased lifespan and ageing-related pathology in these models. Here we demonstrate that transplantation of functional WT stem/progenitor cells isolated from juvenile mice into hosts harbouring dysfunctional MDSPCs leads to a significant extension of healthspan and lifespan ( Fig. 4 ). These results provide experimental evidence that the loss of adult stem cell function directly contributes to ageing-related phenotypes. Interestingly, the function of MDSPCs from aged mice could be restored if they were co-cultured with young WT-MDSPCs ( Fig. 6 ). Similar results were seen in vivo using parabiosis [47] . These observations demonstrate that old, dysfunctional MDSPCs can be rescued by exogenous factors, rather than the cells being inherently defective. This is in contrast to aged haematopoietic stem cells, which appear to have an intrinsic defect (reviewed in ref. 57 ). IP administration of young WT-MDSPCs to progeroid mice promoted growth of the animals, decreased skeletal muscle atrophy, and stimulated neovascularization in the brain and muscle, despite the fact that donor cells were not detected in these tissues ( Figs 4 and 7 ). In addition, transplantation of young WT-MDSPCs directly into progeroid muscle led to muscle regeneration as well as host neovascularization, demonstrating a paracrine mechanism requiring secreted factors ( Fig. 8 ). These observations suggest that the mechanism by which MDSPCs promote healthspan and lifespan extension is likely through the secretion of stimulatory factor(s) that promote regeneration and that cells from old hosts lose this secretory phenotype. This stimulatory factor may be necessary to overcome systemic [48] or local [58] negative regulators of tissue regeneration in aged hosts. Identification of these secreted factors and methods to rejuvenate adult stem cells ex vivo will be critical for regenerative medicine. Our data demonstrate that transplanted MDSPCs can have systemic effects, leading to tissue regeneration in multiple organ systems. Therefore, MDSPCs may have therapeutic value for delaying ageing-related functional decline and treating human progerias. It will be of critical importance to test other adult stem cell types for a similar therapeutic effect. Isolation of MDSPCs All animal experiments were performed with the approval of the University of Pittsburgh Institutional Animal Care and Use Committee. The fraction of slow-adhering cells referred to as MDSPCs were isolated from the skeletal muscle of mice via a modified preplate technique [21] , [22] . Briefly, mouse skeletal muscle is enzymatically digested to a single-cell suspension and the cells are separated by their ability to adhere to collagen-coated flasks. The cells that adhere 2 h post-plating are defined as preplate 1 (pp1, Fig. 2 ). The non-adherent cells (pp2) are transferred to a fresh flask after 24 h. This is repeated five times to isolate the slowly adhering, stem-cell-enriched MDSPC population (pp6 labelled ft). MDSPCs were isolated from young WT (14–21-day-old; f1 C57BL/6:FVB/n or C57BL/10J), adult WT (19-wk-old; f1), old WT (2-yr-old; f1), progeroid Ercc1 −/− (14–21-day-old; f1), Ercc1 −/Δ (19-wk-old; f1) and DNA-repair-deficient Xpa −/− (21-day-old; C57BL/6) mice ( n =3–4 per strain), which were bred at the University of Pittsburgh Division of Laboratory Animal Research. MDSPCs were cultured in proliferation medium (PM): DMEM supplemented with 10% horse serum, 10% fetal bovine serum (FBS), 1% penicillin–streptomycin (all from Invitrogen), and 0.5% chick embryo extract (Accurate Chemical), on collagen-type I-coated flasks. Primary MEFs used for transplantation were prepared from E13–15 day-old embryos and cultured at 3% O 2 (ref. 32 ). To isolate individual clones, 5×10 5 MDSPCs were resuspended in 500 μl media and the FACS Aria cytometer (Becton-Dickinson) was used to place one MDSPC per well in a 96-well collagen-I-coated plate containing 100 μl PM medium. Each well was manually checked to confirm the presence of a single cell. Cells were cultured at 37 °C, 5% CO 2 , in a humidified incubator and medium was changed every 2 days. Proliferation in vitro Cells were plated at a density of 2,000 cells per well in a collagen-type-I–coated 12-well plate. An imaging system (Automated Cell Technologies) equipped with a ×20 objective was used to acquire images at 10-min intervals over a period of 72 h. Forty images at each time point were randomly selected and analysed from three independent experiments on three-to-four distinct cell lines. To estimate PDT, the experimental data sets for each population were curve-fit to the re-arranged Sherley model [38] , [59] , using nonlinear regression to determine the correlation coefficient and dividing fraction for each cell genotype. The division time (DT) of individual cells within the population or of isolated clones was measured by determining the time between cytokinesis events using time-lapsed video recordings (72 h in duration). At least 30 cells were tracked over time in at least 3 MDSPC populations per genotype. For clonal experiments, cells were analysed within 5 days after isolation of clones from pp6. Three-to-four clones were isolated from 2–3 MDSPC populations of each genotype. DT was, therefore, calculated from 6–12 clones per genotype ( Supplementary Table S1 ). Differentiation in vitro To induce myogenic differentiation, MDSPCs were plated at high confluence in PM for 2–3 days then shifted to differentiation medium (DM: DMEM, 2% FBS, 1% penicillin–streptomycin). After 2–3 days, immunostaining for f-MyHC, a marker of terminal myogenic differentiation, was performed. After cold methanol fixation, cells were blocked with 5% goat serum and incubated with f-MyHC mouse monoclonal antibody (1:250; Sigma-Aldrich), secondary biotinylated IgG (1:250; Vector Laboratories) for 1 h, and streptavidin-594 (1:500; Sigma-Aldrich) for 15 min to fluorescently label the myotubes. To visualize the nuclei, the cultures were then incubated with DAPI (4′, 6′ diamidino-2-phyenylindole, 100 ng ml −1 ; Sigma-Aldrich) for 10 min. For negative controls, the primary antibody was omitted or replaced with mouse or rabbit IgG. Fluorescent images were captured and processed using a Leica DMIRB microscope equipped with a QImaging Retiga digital camera both using Northern Eclipse software (v. 6.0; Empix Imaging). We quantified the cells in at least 15 fields each from 3 replica platings of 4 independent experiments. Myogenic differentiation was calculated as the percent of cells (the number of nuclei, detected by DAPI stain) expressing f-MyHC. For adipogenic, osteogenic, and chondrogenic differentiation, MDSPCs were seeded onto 6-well plates and lineage-specific differentiation media (Lonza) was added for 7 days. Expression of lineage-specific markers was measured by reverse transcriptase PCR (rtPCR) as described in Supplementary Methods and Supplementary Table S5 . FACS The preplate technique was utilized to obtain cells from skeletal muscle [21] . Red blood cells were eliminated using a lysis buffer before plating. After 24 h, nonadherent cells in pp3 were collected, centrifuged, resuspended in mouse serum (1:10; Sigma-Aldrich) on ice and counted. Cells were then labelled with rat monoclonal antibodies against CD34, Sca-1, and CD45 conjugated to FITC, PE (both from BD Pharmingen), and APC, respectively (Invitrogen). A separate fraction of each cell pellet was stained with equivalent volumes of isotype control antibodies. Before analysis, 7-amino-actinomycin D (7-AAD) was added for exclusion of nonviable cells. Cells were analysed on a FACSAria cytometer using FACS Diva software, (Becton Dickinson). Sorted gates were defined based on separate cell portions that were labelled with equivalent amounts of appropriately conjugated isotype-matched control antibodies. Positive and negative gates were set by analysing isotype or unstained control samples in each analysis. The average percent of Sca-1 + /CD34 + /CD45 − cells was normalized to pellet weight. To compare differentiation potential, an equal number of sorted cells from each group were plated in 48-well plates and differentiation was induced as described above. Co-culture experiments Ercc1 −/− MDSPCs were plated in the lower compartment of Transwell Permeable Supports (Costar) in PM media at a density of 3,000 cells per well. WT-MDSPCs were seeded into 6.5 mm transwell membrane inserts at the same density in PM media and placed above the ERCC1-deficient MDSPCs. The 24-well plates containing the transwells were then placed in the LCI system for 72 h to acquire time-lapsed images to measure proliferation of the MDSPCs, as described above. As a control, each plate contained wells of Ercc1 −/− MDSPCs without transwell membrane inserts. To measure the differentiation potential of Ercc1 −/− MDSPCs after co-culture, transwell inserts were removed after 72 h and the PM media was switched to DM. After 2–3 days, myogenic differentiation of the cells was tested by immunostaining for f-MyHC, as described above. To quantify differentiation, it was necessary to switch from transwell to conditioned media from young WT-MDSPCs to generate sufficient cells for quantitative immunodetection of myogenic differentiation markers. Young WT-MDSPCs were cultured for 2 days in 25 cm 2 collagen-coated flasks and then treated with differentiation media (DMEM medium supplemented with 2% FBS) for 3 days. The supernatant was collected and used as conditioned media. MDSPCs from 21-day-old Ercc1 −/− mice and 2-yr-old WT mice were grown in the presence of this conditioned media or unconditioned differentiation media to determine the impact on myogenic differentiation. Western blot Three-to-four days after induction of myogenic differentiation, cells were lysed in Laemmli Sample Buffer (Bio-Rad), boiled for 5 min, and centrifuged at 4,000 r.p.m. for 5 min. Each sample was loaded on a 6% SDS-polyacrylamide gel, which was run for 2 h by 100 volts and then transferred for 45 min by 20 volts in a semi-dry transferring apparatus. The membrane was blocked with 5% nonfat dry milk (Bio-rad) in Tris-buffered saline Tween-20 for 1 h and then incubated with mouse anti-MyHC (fast) monoclonal antibody (1:500, Sigma-Aldrich) and mouse anti-β-Actin monoclonal antibody (1:8,000, Sigma-Aldrich), respectively, overnight at 4 °C. After washing 3 times with Tris-buffered saline Tween-20, the membrane was incubated with rabbit anti-mouse IgG (H+L) (1:5,000, Pierce) for 1 h at room temperature. Blots were developed by ECL solution (Pierce). Differences in expression were measured by densitometry using software from SCION Corporation (provided by National Institutes of Health) and reported relative to β-Actin. Tissue staining Microvascular density was measured by co-staining for dystrophin to highlight muscle fibres and CD31 to identify endothelial cells present within microvessels [35] . Briefly, sections of frozen gastrocnemius muscle were formalin fixed, blocked with serum, and incubated with primary antibodies including CD31 (1:250; BD Biosciences) and dystrophin (1:300, Abcam) for 1 h. Goat anti-rat IgG Alexa Fluor 594 (1:300, Invitrogen) and donkey anti-rabbit Alexa Fluor 488 (1:300, Invitrogen) were used to detect CD31 and dystrophin, respectively. DAPI was used to identify cell nuclei. For each image, the total number of muscle fibres and CD31+ cells were counted, and the ratio of CD31+ cells to muscle fibres was reported [35] . To detect nLacZ expression, tissue sections were fixed in 1% glutaraldehyde and incubated with 5-bromo-4-chloro-3-indolyl β-d-galactopyranoside (X-gal) solution for 3 h at 37 °C and counterstained with haematoxylin and/or eosin. For details on co-localizing CD31 and nLacZ staining, see Supplementary Methods . Statistics Statistical analyses were carried out using SigmaStat (Jandel Scientific v2.0) software package. The paired Student's t -test or Mann–Whitney rank sum test was used for direct comparisons between treatment and control groups. For multiple comparisons, the one-way ANOVA or the Kruskal–Wallis one-way ANOVA on ranks was applied. Pairwise multiple comparisons were performed using the Tukey's Test or Dunn's Method following rank-based ANOVA. All values are expressed as the mean±s.d. (or s.e.m. where noted), and P <0.05 was considered significant. How to cite this article: Lavasani, M. et al . Muscle-derived stem/progenitor cell dysfunction limits healthspan and lifespan in a murine progeria model. Nat. Commun. 3:608 doi: 10.1038/ncomms1611 (2012).